Overtemperature-protection intelligent molecular chiroptical photoswitches Stimuli-responsive intelligent molecular machines/devices are of current research interest due to their potential application in minimized devices. Constructing molecular machines/devices capable of accomplishing complex missions is challenging, demanding coalescence of various functions into one molecule. Here we report the construction of intelligent molecular chiroptical photoswitches based on azobenzene-fused bicyclic pillar[ n ]arene derivatives, which we defined as molecular universal joints (MUJs). The Z / E photoisomerization of the azobenzene moiety of MUJs induces rolling in/out conformational switching of the azobenzene-bearing side-ring and consequently leads to planar chirality switching of MUJs. Meanwhile, temperature variation was demonstrated to also cause conformational/chiroptical inversion due to the significant entropy change during the ring-flipping. As a result, photo-induced chiroptical switching could be prohibited when the temperature exceeded an upper limit, demonstrating an intelligent molecular photoswitch having over-temperature protection function, which is in stark contrast to the low-temperature-gating effect commonly encountered. Molecular machines/devices are miniaturized artificial devices, down to nano- to sub-nanoscales, which can accomplish large-amplitude mechanical motions by responding to input stimuli [1] , [2] , [3] . By virtue of an in-depth understanding of molecular motional physics, sophisticated design and organic synthesis, and stimulus-responsive molecular transformations, molecular machines/devices with complex structures and functions have been constructed [4] , such as molecular shuttles [5] , [6] , [7] , [8] , [9] , motors [10] , [11] , [12] , [13] , pumps [14] , [15] , [16] , and elevators [17] . These molecular machines/devices can switch among multi-isomeric states [18] , [19] , [20] by specifically responding to external stimuli, such as solvents [21] , [22] , light [23] , [24] , [25] , [26] , pH [27] , [28] , redox [29] , [30] , [31] , and chemical additives [32] , [33] . Temperature is a universal environmental factor. Unlike the above external stimuli, exerting a thermal effect on a molecular device without affecting its surrounding molecules is difficult. Lowering the temperature could lead to inhibition of some molecular physicochemical pathways, a phenomenon called low-temperature gating [34] . Increasing the temperature generally leads to improved reactivity and conversion pathways, and high-temperature gating has never been observed at the single-molecule level. Therefore, realizing overtemperature protection, which is vital for switching devices/power transistors, such as the stable operation of computers and devices and safety of power supplies, with a molecular device is obviously challenging. Herein, we report an overtemperature-protection function by integrating the thermo- and photoresponsive functions into one pillar[ n ]arene-based bicyclic pseudocatenanes, so-called molecular universal joints (MUJs) [30] , [35] . Azobenzene-bearing MUJ1 and MUJ2 (Fig. 1a ) were synthesized by etherification of a triethylene glycol ether-modified trans -azobenzene derivative with dihydroxylated pillar[6]arene (P[6]) and pillar[5]arene (P[5]) derivatives, respectively, while MUJ3 was obtained by etherification of the tetraethylene glycol ether-modified trans -azobenzene derivative with a dihydroxylated P[6] derivative [30] . The chemical structure of the MUJs was characterized by HR-mass spectrometry and NMR spectroscopic studies. As shown in Fig. 1b , the self-included “ in ” and self-excluded “ out ” conformers of the trans -MUJ enantiomers can interconvert quickly accompanied by the switching of chiral conformers that have clockwise-directed ( R p conformer) and anticlockwise-directed ( S p conformer) arrangement of the substituents, respectively [36] , [37] . However, for cis -MUJ, the large steric hindrance of cis -azobenzene prevents the self-inclusion by the cavity of pillar[6]arene and inhibits the in–out interconversion. Fig. 1: Chemical structures of MUJs and the in–out conformational switching of trans -MUJs. a Chemical structures of MUJ1 , MUJ2 , MUJ3 , G1 , and G2 . b Schematic diagram for the in–out equilibrium of the enantiomers of trans - MUJ1 . Full size image The azobenzene moiety of the MUJs readily underwent cis / trans photoisomerization upon wavelength-selective photoirradiation. trans - MUJ1 showed strong absorption peaks at 294 nm ( ε = 25,896 cm −1 M −1 ) and 365 nm ( ε = 17,093 cm −1 M −1 ), assignable to the transitions of the P[6] and trans -azobenzene moieties, respectively. Photoirradiation at 365 nm led to a rapid decrease in the absorption band at 365 nm (Fig. 2a ) at which the ratio of the absorption spectrum of trans -isomer divided by that of cis -isomer reaches the maximum, accompanied by an increase in the longer wavelength peak at 450 nm due to the transformation to cis -azobenzene. The 1 H-NMR spectral studies indicated that irradiation with a 365 nm LED lamp for 2 min led to a significant upfield shift of proton a of the azobenzene moiety (Fig. 2b ). Meanwhile, proton b of the side ring-bearing hydroquinone unit showed a downfield shift while upfield shift could be observed with protons of several other hydroquinone units (Fig. 2b ), suggesting a significant conformational change from self-included in to self-excluded out conformation upon the trans to cis isomerization, which released the shielding and deshielding effects unequivently exerted on pillar[6]arene subunits. trans -MUJ1 was almost completely converted into cis -MUJ1 in the photostationary state (PSS) under 365 nm photoirradiation (Fig. 3b ). This was also confirmed by HPLC analyses, which gave a cis / trans ratio of 97.8/2.2 in the PSS under 365 nm irradiation (Supplementary Fig. 38 ). 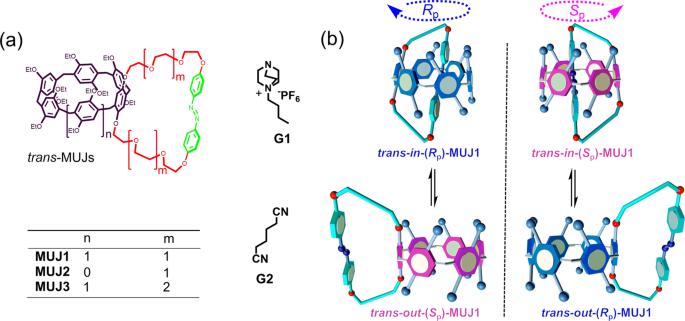Fig. 1: Chemical structures of MUJs and thein–outconformational switching oftrans-MUJs. aChemical structures ofMUJ1,MUJ2,MUJ3,G1, andG2.bSchematic diagram for thein–outequilibrium of the enantiomers oftrans-MUJ1. High cis / trans ratios (>93.5/6.5) were also observed with MUJ2 and MUJ3 (Supplementary Table 1 ) due to the overwhelmingly high absorption of the trans- MUJs at 365 nm. The lifetime of cis isomers of MUJs will be discussed later. Fig. 2: Photoisomerization of MUJ1 by wavelength-selective photoirradiation. a UV-vis absorption spectra of trans - MUJ1 (0.025 mM, chloroform) by alternating irradiation at 365 and 510 nm (xenon grating spectrometer). b 1 H NMR spectra of MUJ1 (2 mM, 400 MHz, rt) in CDCl 3 before (bottom) and after (middle) irradiation at 365 nm for 2 min (LED illuminant) and then after (top) being kept in the dark for 1 week. Full size image Fig. 3: Chiral HPLC spectra and spectrum analysis of the enantiomers of MUJ1 . a Chiral HPLC trace of a mixture containing trans - and cis - MUJ1 (tetrahydrofuran: n -hexane = 1:4, detected at 319 nm). b CD and ( c ) UV-vis spectra of enantiomeric pairs of trans - MUJ1 and cis - MUJ1 measured in the HPLC eluant (tetrahydrofuran: n -hexane = 1:4). Full size image The spectrum of trans- MUJ1 was almost entirely recovered under photoirradiation of cis - MUJ1 at 510 nm (Fig. 2a , Supplementary Fig. 38 ). The trans / cis ratios were in the range of 4.4~12.0 in the PSS at 510 nm. However, the 1 H-NMR spectra of cis- MUJ1 ultimately returned to that of trans- MUJ1 after being kept in the dark for one week (Fig. 2b ), suggesting that trans- MUJ1 is a thermodynamically stable species [38] . Detailed HPLC traces suggested that the complete conversion of cis- MUJ1 to trans- MUJ1 in the dark required more than 66 h at room temperature (Supplementary Fig. 41 ). In contrast, photoirradiation of cis- MUJ1 at 510 nm led to the PSS within several minutes. 1 H-NMR investigation of the photoisomerization between the trans- and cis- MUJs demonstrated that the photoisomerization is reversible and repeatable without destroying the chemical structure of the MUJs (Supplementary Figs. 80 – 82 ). Each trans -MUJ is composed of a pair of isolatable planar chiral enantiomers (Fig. 1b ) [37] , [39] . Successful chiral resolution of all three MUJs was obtained by chiral phase HPLC by using different mobile phases (Supplementary Figs. 35 – 37 ). As illustrated in Fig. 3a , four peaks, corresponding to two pairs of enantiomers of trans - MUJ1 and cis - MUJ1 , were well separated with certain eluent compositions, in which the first and fourth fractions were trans - MUJ1 , and the second and third fractions were cis - MUJ1 . Photoirradiation of the mixture at 365 nm led to an inversion of the relative intensities of the peaks a/d and b/c (Supplementary Fig. S42 ). Circular dichroism (CD) spectra of isolated fractions were measured in the eluate (tetrahydrofuran: n -hexane = 1:4) at room temperature. The four fractions of MUJ1 gave two sets of UV-vis spectra (Fig. 3c ) and two pairs of mirror images in the CD spectra (Fig. 3b ), in agreement with two pairs of enantiomers. The first- and third-eluted fractions of MUJ1 showed positive CD extrema (CD ex ), and the second- and fourth-eluted fractions gave negative CD ex (Fig. 3b ). We have demonstrated that the negative CD ex ca. 310 nm corresponds to the Sp ( Sp , Sp , Sp , Sp , Sp , Sp ) configuration of P[6] derivatives [30] , [35] , and theoretical calculations confirmed that the Sp configuration of P[6] shows a negative CD ex (Supplementary Fig. 157 ). However, since the azobenzene side ring could be either self-included ( in conformer, Fig. 1b ) or self-excluded ( out conformer), the chirality and CD response of the MUJs should critically depend on the conformers they adopt, and therefore, these CD spectral results did not immediately allow for assignment of the absolute configurations of these isomers. Absolute conformation of MUJs Competitive complexation experiments of the MUJs with G1 or G2 were performed to clarify the absolute configurations of the MUJs (Fig. 4a–c ). In chloroform, the weak negative CD ex of the MUJ1 1st fraction (Fig. 4a ) was enhanced upon increasing the concentration of G1 . This suggested that pushing out of the side ring by complexation of G1 led to the S p conformation of the pillar[6]arene core. The 1st fraction of MUJ1 (Fig. 3a ) was thus assigned to be trans -( in-R p / out-S p )- MUJ1 , and the 4th fraction was trans -( in-S p / out-R p )- MUJ1 . Photoisomerization of trans -( in-R p / out-S p )- MUJ1 and trans -( in-S p / out-R p )- MUJ1 led to the 2nd and 3rd fractions, respectively, indicating that the 2nd fraction is cis -( in-R p / out-S p )- MUJ1 and that the 3rd fraction is cis -( in-S p / out-R p )- MUJ1 (Supplementary Fig. 38 ). The absolute configuration of each fraction of MUJ3 was assigned by the same procedure (Fig. 4c ). G1 is too bulky for the cavity of pillar[5]arene, and the absolute configuration of fractions of MUJ2 was assigned based on the complexation experiment with G2 (Fig. 4b ). However, little CD spectral change could be observed with trans- ( in-R p / out-S p )- MUJ2 , even after adding a large excess amount of G2 , suggesting that trans- ( in-R p / out-S p )- MUJ2 almost completely adopts the out conformer (Supplementary Fig. 44 ). Based on the titration experiments (Supplementary Figs. 43 , 45 and 47 ) the association constants K assoc of G1 were determined as (4.9 ± 0.2) × 10 3 M −1 for MUJ1 and (7.5 ± 0.4) × 10 3 M −1 for MUJ3 , respectively, and G2 showed a K assoc of (8.0 ± 0.8) × 10 4 M −1 for MUJ2 . Fig. 4: Solvent effects and competitive complexation of MUJs. CD spectra of trans -( in-R p / out-S p )- MUJ1 ( a ) upon increasing the concentration of G1 in chloroform and ( d ) in different solvents; CD spectra of trans -( in-R p / out-S p )- MUJ2 ( b ) with titrations of G2 in chloroform and ( e ) in different solvents; CD spectra of trans -( in-R p / out-S p )- MUJ3 ( c ) upon increasing the concentration of G1 in chloroform at 25 °C and ( f ) in different solvents. Full size image The CD spectra of the trans -( in-R p / out-S p )-MUJs were measured in various solvents (Fig. 4d–f ), including methanol, acetonitrile, dichloromethane, chloroform, tetrahydrofuran, decahydronaphthalene, and n -hexane. As illustrated in Fig. 4d , the CD spectra of trans- ( in-R p / out-S p )- MUJ1 at room temperature were highly solvent-dependent: CD ex was strongly positive in the solvents n- hexane, decahydronaphthalene, and methanol and weakly positive in acetonitrile or tetrahydrofuran, indicating that a self-included ( in ) conformation dominated in all these solvents. However, CD ex was negative in chloroform or dichloromethane, suggesting that a self-excluded ( out ) conformer was adopted in these two solvents. The solvent-dependent CD spectra of trans- ( in-R p / out-S p )- MUJ3 were similar to those of trans- ( in-R p / out-S p )- MUJ1 (Fig. 4f ). Such solvent effects reflect a delicate interaction balance between the in and out conformers, which involves binding of the solvent molecule(s), self-complexation of the side ring by the pillar[ n ]arene cavity, and solvation of the side ring. In particular, different solvation of the side ring and complexation of solvents by the pillar[ n ]arene cavity should be responsible for this distinct solvent dependence [35] . The strong positive CD ex observed in n- hexane, decahydronaphthalene and methanol should be ascribed to the unfavorable solvation effects of these solvents for the fused azobenzene moiety of MUJ1 and MUJ3 , which facilitated a shift of the in–out equilibrium to form self-complexation conformers. In contrast, the P[5]-based trans- ( in-R p / out-S p )- MUJ2 always presented strong negative CD 310 in all solvents examined, implying that the smaller cavity of P[5] hardly accommodated the azobenzene block of MUJ2 , and the out conformation dominated in different solvents [40] . Furthermore, CD signals of trans -( in - R p / out - S p )- MUJ2 in acetonitrile, dichloromethane, and n -hexane were stronger than in chloroform, decahydronaphthalene, and methanol, presumably due to the strong complexation of the formers with pillar[5]arene which fixes the orientation of each subunit. Light-driven chirality switching of MUJs Trans- ( in-R p / out-S p )- MUJ1 showed a strong positive CD ex in n- hexane at 20 °C due to the self-included in-R p conformation. Photoirradiation of MUJ1 at 365 nm led to a significant decrease in the absorption peak at 365 nm and an increase in the long-wavelength range absorption. Such absorption changes can commonly be used as readouts of azobenzene-based molecular switches. Interestingly, the strong positive CD ex of trans- ( in-R p / out-S p )- MUJ1 decreased and inverted to a strong negative CD signal upon irradiation at 365 nm, and the weak CD signal peak at 435 nm significantly increased. Moreover, the original CD spectrum could be recovered by photoirradiation at 510 nm, at which the ratio of the absorption spectrum of cis- isomer divided by that of trans- isomer reaches the maximum (Fig. 6a and Supplementary Figs. 54 – 67 ). No fatigue was observed for the light-driven planar chirality switching between trans-in- ( R p )- MUJ1 and cis-out- ( S p )- MUJ1 after several tens of cycles (Fig. 6b ). Such a CD spectral change indicated a switching from trans-in- ( R p )- MUJ1 to cis-out- ( S p )- MUJ1 , demonstrating that the planar chirality of MUJ1 can be switched by changing the irradiation wavelength. Such a photoinduced CD spectral change provides a powerful chiroptical switch that allows for distinctively determining on/off based on the positive/negative sign of CD ex rather than on the intensity, as commonly encountered in absorption and emission spectroscopic techniques. The rolling out of the side ring upon the trans to cis isomerization seems reasonable because the cis- azobenzene block became too bulky to be accommodated in the cavity of P[6], i.e., the trans- azobenzene block preferred to be included in the cavity, while it was excluded upon conversion to the cis- configuration (Fig. 5 ). Alternating photoirradiation of trans- ( in-R p / out-S p )- MUJ1 at 365 nm and 510 nm led to reversible switching of both the CD (anisotropy factor g = Δ ε / ε , where ε is the molar extinction coefficient at a particular wavelength, Fig. 6b ) and UV-vis (Supplementary Figs. 56 – 67 ) spectra between their PSSs. Fig. 5: Light-driven chirality switching of ( in-R p / out-S p )- MUJ1 . Suppositional mechanism of light-driven chirality switching of ( in-R p / out-S p )- MUJ1 . Full size image Fig. 6: CD spectral change of the enantiomers of MUJs upon selective wavelength photoirradiation. a CD spectra and ( b ) extremum changes (~310 nm) of the anisotropy factor ( g ) of trans -( in-R p / out-S p )- MUJ1 upon alternating irradiation at 365 nm (blue signet) and 510 nm (red signet, xenon light source) in n -hexane. CD spectra of ( c ) trans -( in-R p / out-S p )- MUJ2 and ( d ) trans -( in-R p / out-S p )- MUJ3 upon alternating irradiation at 365 and 510 nm in n -hexane. Full size image In contrast, trans- ( in-R p / out-S p )- MUJ2 showed a strong negative CD ex in n- hexane at room temperature, suggesting that the trans -azobenzene moiety was located outside the P[5] cavity, which could be ascribed to the azobenzene moiety being too bulky to be comfortably accommodated by the P[5] cavity [41] . Photoirradiation of trans- ( in-R p / out-S p )- MUJ2 at 365 nm led to a significant decrease and almost inversion in CD ex (Fig. 6c and Supplementary Figs. 68 – 69 ), suggesting that the out reference became weaker. Molecular model studies of trans - MUJ2 suggested that the side ring is stretched flat and is relatively rigid (Supplementary Fig. 84 ) due to the long strip structure of azobenzene, which prevents even partial inclusion of the side ring by the small pillar[5]arene cavity. However, the side ring in cis - MUJ2 is much more flexible, which allows the triethylene glycol ether chain to be partially included in the P[5] cavity [35] (Supplementary Figs. 85 – 86 ). Indeed, 1 H-NMR spectra of MUJ2 recorded after 365 nm irradiation showed significantly upfield-shifted protons of the triethylene glycol ether chain, demonstrating self-inclusion of the fused glycol ether once trans - MUJ2 transformed to cis - MUJ2 (Supplementary Fig. 81 ). However, the cis- azobenzene block is too bulky for the P[5] cavity, which prevents complete chirality switching to the self-included conformer. The decreased negative CD ex caused by irradiation at 365 nm almost completely recovered to the initial state after irradiation at 510 nm (Fig. 6c and Supplementary Figs. 68 – 69 ). Trans- ( in-R p / out-S p )- MUJ3 , which has a longer glycol ether chain and therefore a more flexible side ring than trans- ( in-R p / out-S p )- MUJ1 , also showed a strong positive CD ex (Fig. 6d ) in n- hexane, suggesting that the trans- azobenzene block of MUJ3 was self-included in the cavity. However, unlike the chiroptical inversion observed with MUJ1 , the positive CD ex of MUJ3 was significantly decreased under irradiation at 365 nm and recovered with irradiation at 510 nm. This phenomenon suggested that the side ring of MUJ3 was only partially excluded from the pillar[6]arene cavity when transformed to cis- azobenzene (Supplementary Figs. 72 – 75 ). We ascribed this to the more flexible side ring of MUJ3 , which allows the glycol ether chain to be partially self-accommodated in the P[6] cavity when the trans -azobenzene isomerizes to the cis -azobenzene, thus hampering the chirality switching of trans- ( in-R p / out-S p )- MUJ3 . The above result indicated that the steric effect was critically affected by the cavity size and the chain length in the present system, and appropriate size matching between the cavity and the side ring as well as the rigidity of the side rings is pivotal to the light-driven chirality switching behavior. Interestingly, the light-driven chirality switching of trans- ( in-R p / out-S p )- MUJ1 could also be observed in the coating film. A film of trans- ( in-R p / out-S p )- MUJ1 was prepared by spin-coating and then kept under vacuum to dry for 24 h. The film showed the strong positive CD ex of trans- ( in-R p / out-S p )- MUJ1 , which changed to a strong negative CD ex when irradiated at 365 nm but recovered to the positive CD ex under irradiation at 510 nm (Fig. 7a ). The reversible light-driven chirality switching of trans- ( in-R p / out-S p )- MUJ1 could be repeated many times (Fig. 7b ), indicating that the trans / cis isomerization of the azobenzene block can effectively trigger mechanical rolling in/out of the side ring [42] . Such light-driven planar chirality switching of the unimolecular system in the coating film makes MUJ1 a promising candidate for photoresponsive switch materials. Fig. 7: Light-driven chirality switching of ( in-R p / out-S p )- MUJ1 in the coating film. a CD spectra of the spin-coated film of trans -( in-R p / out-S p )- MUJ1 under alternating irradiation at 365 and 510 nm (xenon light source). b Extremum changes (~310 nm) of the anisotropy factor g of trans-( in-R p / out-S p )- MUJ1 upon alternating irradiation at 365 nm (blue signet) and 510 nm (red signet). Full size image Overtemperature protection for light-driven chirality switching Self-sensing and a feedback ability for temperature perturbances are critically important for intelligent microdevices, having potential applications in, for example, microenvironment temperature sensing and overtemperature protection of microcircuits. While inhibition of certain molecular chemical and physical processes by reducing the temperature is an often-observed phenomenon, inhibiting on/off molecular switching by increasing the temperature is challenging, particularly at the single-molecule level. Variable temperature CD (VT CD) spectra of trans- ( in-R p / out-S p )-MUJs were examined in various solvents (Supplementary Figs. 87 – 107 ). Increasing the temperature led to a decrease in the CD ex of trans- ( in-R p / out-S p )- MUJ2 in all solvents examined (Fig. 8b and Supplementary Figs. 94 – 100 ), indicating that the out conformer trans-out- ( S p )- MUJ2 was the main conformer in the temperature range examined. However, the CD spectra of trans- ( in-R p / out-S p )- MUJ1 and trans- ( in-R p / out-S p )- MUJ3 exhibited significant temperature dependence. For trans- ( in-R p / out-S p )- MUJ1 , as an example, the negative CD ex in tetrahydrofuran at 50 °C was reduced upon decreasing the temperature and finally inverted to give a positive CD ex at 5 °C (Fig. 8a ), demonstrating a conformational transformation from trans - out- ( S p ) - MUJ1 to trans - in- ( R p ) - MUJ1 . The UV-vis spectra of the trans -MUJs were hardly changed by the temperature variation (Supplementary Figs. 87 – 107 ), indicating no trans to cis isomerization of the azobenzene blocks with the temperature variation. Raising the temperature back to 50 °C led to a complete recovery of the initial CD spectrum of trans- ( in-R p / out-S p )- MUJ1 . The in conformer is favored at low temperatures, which seems reasonable because the in conformer should be stabilized by van der Waals contact, C–H…O, π−π, and dipole–dipole interactions between the P[6] cavity and the side ring but is entropy disfavored due to the loss of the motional and rotational freedom of both the side ring and P[6] units. Temperature-driven chirality inversions were observed in tetrahydrofuran, chloroform, dichloromethane, and acetonitrile for MUJ1 (Fig. 8a and Supplementary Figs. 90 – 92 ) and in tetrahydrofuran and acetonitrile for MUJ3 (Fig. 8c and Supplementary Fig. 106 ). Such temperature-driven chiroptical switching demonstrated a delicate dynamic balance established by the significant entropy differences between the in and out conformers. It, therefore, provided a powerful tool to regulate the on/off switching of the MUJs and to implement sensing and feedback of microenvironmental temperature perturbances. Based on the VT CD spectral changes [43] , the entropy (ΔΔ S ) and enthalpy (ΔΔ H ) changes for the in / out conformational switching of MUJ1 in CHCl 3 were estimated as −16.5 J mol −1 K −1 and −4.5 KJ mol −1 , respectively. This demonstrates that the out -to- in conformational switching is enthalpically favorable but disfavored entropically. Fig. 8: Variable temperature CD spectra of the enantiomers of MUJs. VT CD spectra of ( a ) trans -( in-R p / out-S p )- MUJ1 , ( b ) trans -( in-R p / out-S p )- MUJ2 , and ( c ) trans -( in-R p / out-S p )- MUJ3 in tetrahydrofuran at 5 °C (black line), 15 °C (red line), 25 °C (blue line) 35 °C (magenta line) and 50 °C (green line), respectively. Full size image The unique temperature and light dual-responsive property of MUJ1 endow it with the potential to serve as a temperature-responsive molecular photoswitch. Irradiating trans- ( in-R p / out-S p )- MUJ1 at −2 °C with light at 365 and 510 nm caused definite CD ex sign inversion (Fig. 9a ), demonstrating the operation of light-driven switching. However, at 55 °C, trans- ( in-R p / out-S p )- MUJ1 consistently showed a negative CD ex upon irradiation at both 365 and 510 nm (Fig. 9a ), indicating silencing of the chirality inversion at high temperatures. Detailed investigation of the temperature-dependent photoswitching behavior (Fig. 9a ) revealed a critical temperature T 0 of 30.3 °C (Fig. 9b ), below which CD ex exhibited positive/negative switching upon alternating photoirradiation with light at 365 nm and 510 nm and above which CD ex consistently exhibited a negative sign regardless of the irradiation wavelength employed. 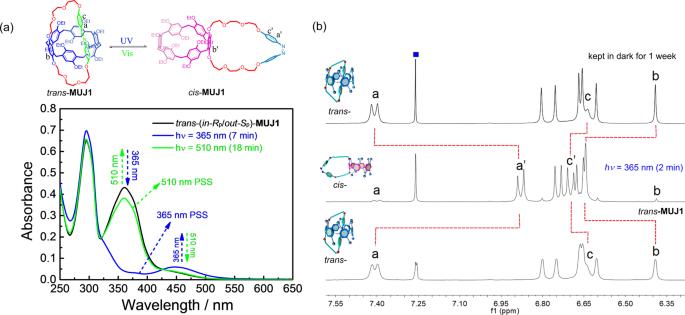Fig. 2: Photoisomerization ofMUJ1by wavelength-selective photoirradiation. aUV-vis absorption spectra oftrans-MUJ1(0.025 mM, chloroform) by alternating irradiation at 365 and 510 nm (xenon grating spectrometer).b1H NMR spectra ofMUJ1(2 mM, 400 MHz, rt) in CDCl3before (bottom) and after (middle) irradiation at 365 nm for 2 min (LED illuminant) and then after (top) being kept in the dark for 1 week. Therefore, the VT CD spectra of ( in-R p / out-S p )- MUJ1 in the PSS at 365 nm were investigated (Supplementary Figs. 113 – 118 ) to gain insight into the temperature-regulated light-driven chirality switching. As shown in Fig. 9b , ( in-R p / out-S p )- MUJ1 in the PSS at 365 nm presented a consistent negative g factor in all of the examined temperature regime, while ( in-R p / out-S p )- MUJ1 in the PSS at 510 nm presented a positive g factor in the low-temperature regime ( T < 30.3 °C) and a negative g factor in the high-temperature regime ( T > 30.3 °C). This phenomenon indicated that temperature can serve as an effective external stimulus to regulate the light-driven chirality switching of ( in-R p / out-S p )- MUJ1 , which can be switched on by cooling and off by heating. As discussed above, the regulatory mechanism should be achieved by the synergistic effects between the two independent mechanisms, i.e., the temperature-regulated in–out equilibrium and the light-controlled photoisomerization of the azobenzene block (Supplementary Fig. 156 ). Fig. 9: Temperature regulation of the light-driven CD spectral inversion of enantiomeric MUJ1 . a VT CD spectra of ( in-R p / out-S p )- MUJ1 in the PSS at 365 nm (blue line) and 510 nm (red, magenta, and pink lines) in tetrahydrofuran. The CD spectra of ( in-R p / out-S p )- MUJ1 with positive CD extrema (CD ex ) at ca. 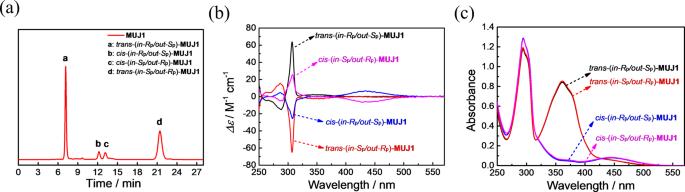Fig. 3: Chiral HPLC spectra and spectrum analysis of the enantiomers ofMUJ1. aChiral HPLC trace of a mixture containingtrans- andcis-MUJ1(tetrahydrofuran:n-hexane = 1:4, detected at 319 nm).bCD and (c) UV-vis spectra of enantiomeric pairs oftrans-MUJ1andcis-MUJ1measured in the HPLC eluant (tetrahydrofuran:n-hexane = 1:4). 310 nm is shown as the red line, while that with negative CD ex is shown as the pink line and that between the two is shown as the magenta line. b VT anisotropy factor changes at 308 nm of ( in-R p / out-S p )- MUJ1 in the PSS at 365 nm (diamond) and 510 nm (circle) in tetrahydrofuran. 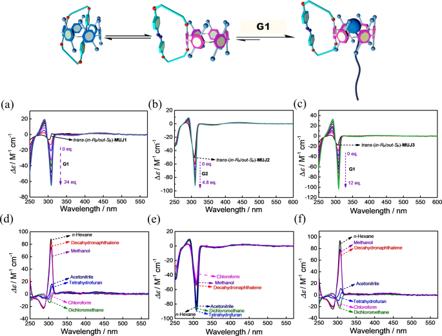Fig. 4: Solvent effects and competitive complexation of MUJs. CD spectra oftrans-(in-Rp/out-Sp)-MUJ1(a) upon increasing the concentration ofG1in chloroform and (d) in different solvents; CD spectra oftrans-(in-Rp/out-Sp)-MUJ2(b) with titrations ofG2in chloroform and (e) in different solvents; CD spectra oftrans-(in-Rp/out-Sp)-MUJ3(c) upon increasing the concentration ofG1in chloroform at 25 °C and (f) in different solvents. The blue signet presenting a negative g factor and the red signet presenting a positive g factor. Full size image Adjustable critical temperature of switching Furthermore, the critical temperature ( T 0 ) for the regulation of the light-driven chirality switching can be adjusted by changing the solvents or solvent composition (Table 1 ). For example, the critical temperature T 0 was improved to 47.6 °C in acetonitrile but decreased to 29.7 °C in chloroform. Moreover, by using a mixture of acetonitrile and tetrahydrofuran as a solvent, T 0 could be conveniently adjusted from 8.8 to 34 °C simply by changing the solvent composition. This unambiguously expands the application domains and improves the regulatory capabilities of the intelligent chirality switch. Table 1 Critical temperature ( T 0 ) of ( in-R p / out-S p )- MUJ1 in different solvents. Full size table In summary, we demonstrated an intelligent molecular switch that shows a temperature- and photoresponsive on/off switch function. Such orthogonal control allows photoinduced rolling in/out and chiroptical switching to be prohibited when the temperature exceeds an upper limit, realizing overtemperature-protection intelligent molecular photoswitches. The upper-temperature limit could be conveniently adjusted by manipulating the solvent composition. This study realized the challenging high-temperature-gating effect at the molecular level and represents a prominent step forward for constructing an intelligent molecular machine/device capable of performing complex functions. A Chiralpak IA column was used for chiral separation. The 365 and 510 nm light sources for photoresponsive CD spectral measurement were used with a grating spectrometer on a JASCO FP 8500 fluorescence spectrometer. A 365 nm LED spot curing system was used for photoresponsive 1 H-NMR measurements. CD spectra were recorded as θ in millidegrees. The anisotropy factor g was calculated using the equation g = Δ ε / ε , where ε is the molar extinction coefficient at a particular wavelength. 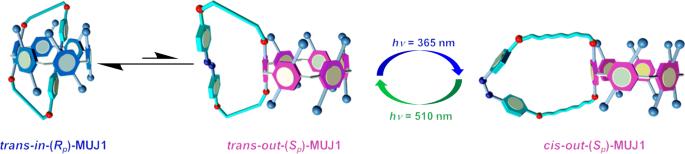Fig. 5: Light-driven chirality switching of (in-Rp/out-Sp)-MUJ1. Suppositional mechanism of light-driven chirality switching of (in-Rp/out-Sp)-MUJ1. 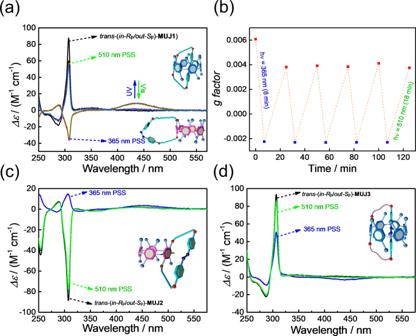Fig. 6: CD spectral change of the enantiomers of MUJs upon selective wavelength photoirradiation. aCD spectra and (b) extremum changes (~310 nm) of the anisotropy factor (g) oftrans-(in-Rp/out-Sp)-MUJ1upon alternating irradiation at 365 nm (blue signet) and 510 nm (red signet, xenon light source) inn-hexane. CD spectra of (c)trans-(in-Rp/out-Sp)-MUJ2and (d)trans-(in-Rp/out-Sp)-MUJ3upon alternating irradiation at 365 and 510 nm inn-hexane. 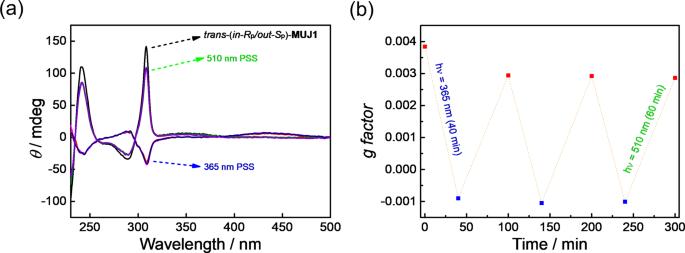Fig. 7: Light-driven chirality switching of (in-Rp/out-Sp)-MUJ1in the coating film. aCD spectra of the spin-coated film oftrans-(in-Rp/out-Sp)-MUJ1under alternating irradiation at 365 and 510 nm (xenon light source).bExtremum changes (~310 nm) of the anisotropy factor g of trans-(in-Rp/out-Sp)-MUJ1upon alternating irradiation at 365 nm (blue signet) and 510 nm (red signet). 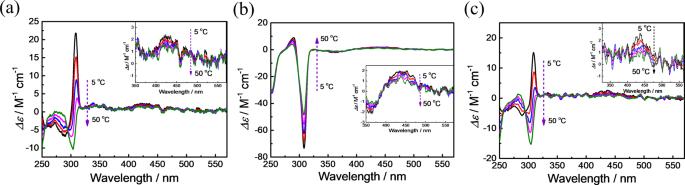Fig. 8: Variable temperature CD spectra of the enantiomers of MUJs. VT CD spectra of (a)trans-(in-Rp/out-Sp)-MUJ1, (b)trans-(in-Rp/out-Sp)-MUJ2, and (c)trans-(in-Rp/out-Sp)-MUJ3in tetrahydrofuran at 5 °C (black line), 15 °C (red line), 25 °C (blue line) 35 °C (magenta line) and 50 °C (green line), respectively. 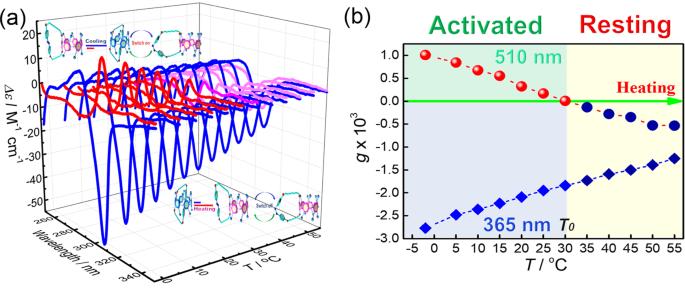Fig. 9: Temperature regulation of the light-driven CD spectral inversion of enantiomericMUJ1. aVT CD spectra of (in-Rp/out-Sp)-MUJ1in the PSS at 365 nm (blue line) and 510 nm (red, magenta, and pink lines) in tetrahydrofuran. The CD spectra of (in-Rp/out-Sp)-MUJ1with positive CD extrema (CDex) at ca. 310 nm is shown as the red line, while that with negative CDexis shown as the pink line and that between the two is shown as the magenta line.bVT anisotropy factor changes at 308 nm of (in-Rp/out-Sp)-MUJ1in the PSS at 365 nm (diamond) and 510 nm (circle) in tetrahydrofuran. The blue signet presenting a negativegfactor and the red signet presenting a positivegfactor. The molar ellipticity was obtained by the formula Δ ε = θ /32980 cl , where l is in cm.